Genome sequence of mungbean and insights into evolution withinVignaspecies Mungbean ( Vigna radiata ) is a fast-growing, warm-season legume crop that is primarily cultivated in developing countries of Asia. Here we construct a draft genome sequence of mungbean to facilitate genome research into the subgenus Ceratotropis , which includes several important dietary legumes in Asia, and to enable a better understanding of the evolution of leguminous species. Based on the de novo assembly of additional wild mungbean species, the divergence of what was eventually domesticated and the sampled wild mungbean species appears to have predated domestication. Moreover, the de novo assembly of a tetraploid Vigna species ( V. reflexo-pilosa var. glabra ) provides genomic evidence of a recent allopolyploid event. The species tree is constructed using de novo RNA-seq assemblies of 22 accessions of 18 Vigna species and protein sets of Glycine max . The present assembly of V. radiata var. radiata will facilitate genome research and accelerate molecular breeding of the subgenus Ceratotropis . Mungbean ( Vigna radiata (L.) R. Wilczek) is a fast-growing warm-season legume species belonging to the papilionoid subfamily of the Fabaceae and has a diploid chromosome number of 2 n =2 x =22. Mungbean is cultivated mostly in South, East and Southeast Asia by small holder farmers for its edible seeds and sprouts. Mungbean seeds are a good source of dietary protein and contain higher levels of folate and iron than most other legumes [1] . Moreover, mungbean, as a legume crop, fixes atmospheric nitrogen via root rhizobial symbiosis, leading to improved soil fertility and texture [2] . Intercropping mungbean in rice–rice and rice–wheat systems increases the yield of the subsequent cereal crop and reduces pest incidence [3] , [4] . Genetic diversity data and archaeological evidence suggest that mungbean was domesticated in India [5] . India is also the world’s largest producer of mungbean, accounting for over 50% of the global annual production (~6 million tons), followed by China and Myanmar [6] . In spite of its economic importance genomics of mungbean has not been intensively studied. Whole-genome sequences have become available for several legumes, such as Medicago truncatula , Cicer arietinum , Lotus japonicus , Glycine max and Cajanus cajan , whereas the genomic resources for mungbean remain scarce [7] , [8] , [9] , [10] , [11] . Along with mungbean, the subgenus Ceratotropis of genus Vigna contains several major agriculturally important legumes, including créole bean ( V. reflexo - pilosa var. glabra ), black gram ( V. mungo ), rice bean ( V. umbellata ), moth bean ( V. aconitifolia ) and adzuki bean ( V. angularis ). The genome sizes of Vigna species are highly variable, ranging from 416 to 1,394 Mb (refs 12 , 13 ). Most Vigna species are diploid, whereas V. reflexo-pilosa is tetraploid (2 n =4 x =44; ref. 14 ). Genome expansion and polyploidization are considered major mechanisms of plant speciation, but the effects of polyploidy on species evolution still remain unclear [15] . With the availability of modern genomics tools, traces of allopolyploidization can be tracked down which will further provide insights into adaption and speciation [16] . In the present study, we construct a draft genome of the cultivated mungbean ( V. radiata var. radiata VC1973A ) on a chromosomal scale. For detailed understanding of domestication, polyploidization and speciation in the genus Vigna , whole-genome sequences of a wild relative mungbean ( V. radiata var. sublobata ) and of a tetraploid relative of mungbean ( V. reflexo-pilosa var. glabra ), as well as transcriptome sequences of 22 Vigna accessions of 18 species are produced. Because of its short life cycle and small genome size, Vigna species may be used as model legume plants in genetic research to shed light on crop domestication and species divergence. Most importantly, the mungbean whole-genome sequence information produced by this study will boost genomics research in Vigna species and accelerate mungbean breeding programmes, which can be a potential framework for future resequencing efforts of the Vigna germplasms. Genome assembly We sequenced domesticated V. radiata var. radiata (2 n =2 x =22), its polyploid relative V. reflexo-pilosa var. glabra (2 n =4 x =44), and its wild relative V. radiata var. sublobata (2 n =2 x =22). For V . radiata var. radiata , the pure line VC1973A was chosen for genome sequencing. VC1973A was developed at the AVRDC-The World Vegetable Center in 1982; since then, it has been widely grown in Korea, Thailand, Taiwan, Canada and China as a heteronymous cultivar called ‘Seonhwanogdu’ in Korea, ‘Kamphaeng Saen 1’ in Thailand and ‘Zhong Lu’ in China. A high-quality draft genome sequence of the diploid V. radiata var. radiata VC1973A (2 n =2 x =22) with an estimated genome size of 579 Mb (1.2 pg per 2C) was constructed [17] . We prepared five libraries for sequencing by Illumina HiSeq2000 including 180 and 500 bp paired-end libraries and 5, 10 and 40 kb mate-pair libraries. 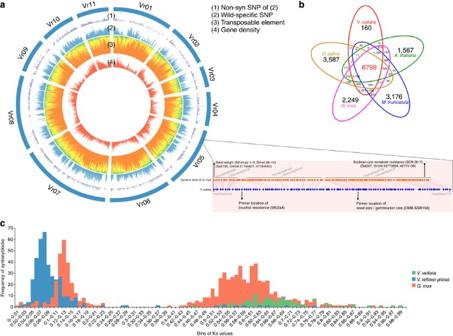Figure 1: Summary of thede novogenome assembly and sequencing analysis of mungbean. (a) SNP distributions between domesticated and wild mungbeans are depicted in the outer circle of the circular map. The middle circle represents the proportions of repeated elements including LTR/Gypsy (orange), LTR/Copia (yellow), LINE (blue) and DNA transposons (green). The inner circle shows gene densities across the chromosomes. On Vr05, two QTL locations were identified at the outermost layer, and they were consistent withG. maxQTLs based on the syntenic relationship, as described schematically. (b) An OrthoMCL clustering analysis of five gene sets fromA. thaliana,M. truncatula,G. max,O. sativaandV. radiata. Each value within Venn diagram shows the number of orthologue/paralogue clusters. (c) Frequency distribution of Ks values inV. radiata(red),V. reflexo-pilosa(sky blue) andG. max(green). These libraries provided a 320-fold base pair coverage of the estimated genome size ( Supplementary Table 1 ). In addition, long reads providing approximately fivefold genome coverage were produced by sequencing using GS FLX+. The short reads were assembled using ALLPATHS-LG software [18] , producing 2,800 scaffolds with an N50 length of 1,507 kb. The total length of the scaffolds was ~431 Mb. The long reads generated by GS FLX+ were assembled into 180,372 contigs using Newbler 2.5.3 software. In total, 144,213 of the GS FLX contigs were consistent with the scaffolds from ALLPATHS-LG. 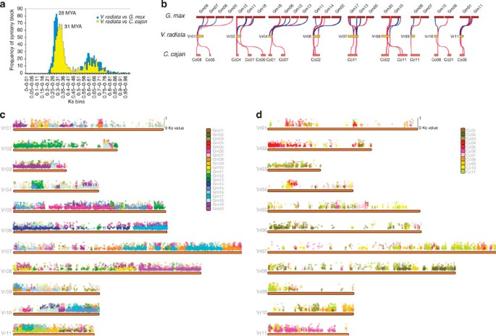Figure 2: Analysis of syntenic relationships in legumes within the millettioid clade. (a) Estimation of divergence times betweenV. radiataandC. cajan, and betweenV. radiataandG. max. (b) Visualization of chromosomal rearrangements amongV. radiatavar.radiata,G. maxandC. cajan. Chromosomes amongV. radiatavar.radiata,C. cajanandG. max(A genome) are connected by red lines, and chromosomes betweenV. radiatavar.radiataandG. max(B genome) are linked by blue lines. (c) Syntenic relationship betweenV. radiataandG. max; thex-axis indicates chromosomal locations and they-axis indicates Ks value. Each dot represents the location of a synteny block with its Ks median value, showing both conservation and chromosomal rearrangements of syntenic blocks. (d) Depiction of the syntenic relationship betweenV. radiataandC. cajan. The non-matched GS FLX+ contigs were divided into 5 kb pseudo-mate-pair reads and assembled using ALLPATHS-LG software to improve the quality of the assembly, resulting in 2,748 scaffolds with an N50 length of 1.52 Mb ( Supplementary Table 2 ). The total length of the produced scaffolds was 431 Mb, representing 80% of the genome size of 543 Mb estimated from 25-base kmer frequency distribution ( Supplementary Fig. 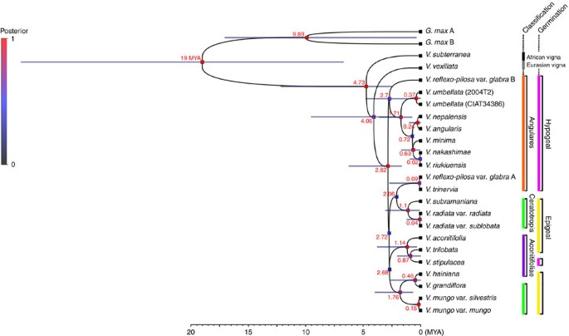Figure 3: Species tree for 22Vignaaccessions and close legume relative,G. max. Average divergence dates were depicted for the nodes estimated by a Bayesian MCMC method. The horizontal bars represent the 95% highest posterior density (HPD) interval at each node estimated by tested genes. The colour of the square on each node represents the posterior probability according to colour gradation from black (0) through blue (0.5) to red (1). The root divergence time was set to a 19 MYA betweenV. radiatavar.radiataandG. maxfollowing the estimation of Lavinet al.27 1 ) ( Supplementary Table 3 ) ( Fig. 1a ). Figure 1: Summary of the de novo genome assembly and sequencing analysis of mungbean. ( a ) SNP distributions between domesticated and wild mungbeans are depicted in the outer circle of the circular map. The middle circle represents the proportions of repeated elements including LTR/Gypsy (orange), LTR/Copia (yellow), LINE (blue) and DNA transposons (green). The inner circle shows gene densities across the chromosomes. On Vr05, two QTL locations were identified at the outermost layer, and they were consistent with G. max QTLs based on the syntenic relationship, as described schematically. ( b ) An OrthoMCL clustering analysis of five gene sets from A. thaliana , M. truncatula , G. max , O. sativa and V. radiata . Each value within Venn diagram shows the number of orthologue/paralogue clusters. ( c ) Frequency distribution of Ks values in V. radiata (red), V. reflexo-pilosa (sky blue) and G. max (green). Full size image We constructed a mungbean genetic map from a F 6 population of 190 recombinant inbred lines (RILs) generated by single-seed descent from a cross between VC1973A and the Korean landrace V2984 ( V. radiata var. radiata ) through genotyping-by-sequencing (GBS). Of 1,993 single nucleotide polymorphisms (SNPs), 1,321 (covering 11 linkage groups) were used to construct a genetic map ( Supplementary Fig. 2 ). In total, 239 scaffolds could be anchored to the genetic map through these SNPs; however, 86 scaffolds remained unoriented because only a single SNP was available to anchor these scaffolds on the genetic map. The resulting pseudochromosomes representing 11 linkage groups had an N50 length of 35.4 Mb and covered 314 Mb, corresponding to 73% of the total assembled sequences. In addition to VC1973A , we sequenced a wild relative ( V. radiata var. sublobata , accession TC1966 ) of domesticated V. radiata var. radiata . Two types of libraries, a 180 bp paired-end and a 5 kb mate-pair library, produced 8,161 scaffolds with an N50 length of 214 kb, covering 423 Mb and corresponding to ~84% of the estimated genome size of 501 Mb ( Supplementary Table 3 ). A tetraploid relative, V. reflexo-pilosa var. glabra , accession V1160, was also sequenced using 180 bp pair-end and 5 kb mate-pair libraries. The resulting assembly consisted of 29,166 scaffolds with a N50 length of 63 kb, covering 792 Mb. The distribution of the kmer frequency led to an estimated genome size of 968 Mb, which was almost twice the size of the mungbean genome. Thus, ~82% of the whole genome of the tetraploid Vigna species was captured by the sequencing effort. Repetitive sequences and transposable elements In plants, transposable elements are a major driver of genome expansion. Homology- and structure-based surveys have revealed that repetitive sequences occupy ~50.1% of the mungbean genome ( Fig. 1a ). Long terminal repeat (LTR) retrotransposons are the predominant class of transposable elements in the mungbean genome, consistent with other legume species [7] , [8] , [9] , [10] , [11] . 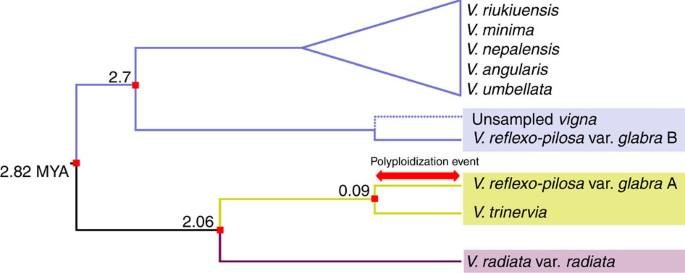Figure 4: Schematic illustration of allopolyploidization history of theV. reflexo-pilosavar.glabra. Red arrow indicates the putative date (maximum 0.09 MYA) of polyploidization event ofV. reflexo-pilosavar.glabra. The number at each node represents the divergence time estimated by a Bayesian MCMC method. We determined that 25.2% of the mungbean genome consisted of LTR/Gypsy, and 11.3% consisted of LTR/Copia type elements ( Supplementary Table 4 ) [19] , [20] , [21] . In contrast, class II DNA transposons, including CACTA, Mutator, PIF-Harbinger, hAT, Helitron, MULE-MuDR and Tc1-Mariner, accounted for ~2.5% of the mungbean genome. The proportion of Mutator was the highest (1.4%), and Tc1-Mariner was the lowest (0.02%). Genome characterization and gene annotation Genes were predicted and annotated from the repeat-masked mungbean genome sequence. We performed de novo and homology-based gene predictions using the Maker [22] pipeline based on data from the RNA-seq assemblies of four different tissues: leaf, flower, pod and root ( Supplementary Tables 5 and 6 ). The predicted mungbean proteins represented a 97% match to the set of 248 eukaryotic core proteins proposed to assess the completeness of the genome sequence ( Supplementary Table 3 ) [23] . The sequence length distributions of the genes, exons, coding DNA sequences (CDS) and introns by plant species showed high consistency among Arabidopsis thaliana , soybean and mungbean, indicating that our gene predictions were highly reliable ( Supplementary Fig. 3 ). In total, 22,427 genes were identified with high confidence, and 18,378 genes were located on pseudochromosomes ( Fig. 1a ). The 22,427 protein sets of V. radiata var. radiata and the protein sequences of A. thaliana , M. truncatula , Oryza sativa and G. max were compared by software OrthoMCL [24] . There were a total of 6,799 gene clusters shared in all five species, and 160 clusters were composed of only V. radiata var. radiata proteins ( Fig. 1b ). We assigned annotations to these proteins using Interproscan [25] and BLAST against Arabidopsis proteins ( Supplementary Data 1 ). In addition, we predicted 2,310 non-coding genes, including 629 transfer RNAs, 280 ribosomal RNAs, 537 microRNAs, 717 small nucleolar RNAs, 110 small nuclear RNAs and 37 other regulatory RNAs ( Supplementary Table 7 ). In total, 1,850 genes encoding transcription factors (TFs) were identified in the mungbean genome by Pfam annotation, and the relative TF abundance was compared with that of other plant genomes ( Supplementary Table 8 ). The overall distribution of TF genes in each genome was highly consistent among the plant genomes ( Supplementary Fig. 4 ). The most highly represented TF family was MYB, followed by AP2/EREBP and bHLH. Notably, the bZIP2 family accounted for <1% of the total TFs in legume genomes compared with those of non-legume genomes, A. thaliana , Zea mays , O. sativa and Brachypodium distachyon, in which bZIP2 represented >3%. Thus there was most likely a reduction in this specific TF family in a common ancestor of these legume genomes. Domestication of mungbean Crops have undergone domestication through selective breeding to acquire traits that are beneficial for their use by humans. The relationship between the genomes of VC1973A and its wild relative ( V. radiata var. sublobata ) TC1966 can serve as a model to understand mungbean domestication. The paired-end short reads derived from TC1966 and an additional domesticated landrace, V2984 , were mapped against the V. radiata var. radiata genome ( Supplementary Table 1 ). The mapped regions spanned 401 and 422 Mb, representing 93 and 98% coverage of the V. radiata var. radiata genome sequence, respectively. In total, 2,922,833 SNPs supported by at least five reads were found between domesticated and wild mungbean, corresponding to a SNP frequency of 6.78 per 1 kb. Of the 63,294 SNPs detected in the CDS regions, 30,405 were non-synonymous, accounting for a total of 10,641 genes ( Supplementary Table 9 ). Out of 342,853 total INDELs, 55,689 were located within the genic boundaries, including 576 deletions and 526 insertions that were predicted to cause frameshift mutations in 551 and 506 genes, respectively. Among the domesticated mungbeans, 775,831 high-confidence SNPs at a frequency of 1.8 SNPs per 1 kb, including 98,590 INDELs, were identified. Of the total 19,541 SNPs in the CDS regions, 9,378 were found to be non-synonymous and affected a total of 3,233 genes. In total, 235,641,385 bases were conserved among all three genotypes. There were 2,425,069 bases conserved between the domesticated mungbeans, which were exclusively polymorphic between VC1973A and TC1966 . Of the 51,351 wild-genotype-specific mungbean SNPs in CDS, 24,599 were non-synonymous where they were distributed over 9,344 genes ( Fig. 1a ). Any protein changes underlying phenotypic differences between domesticated and wild mungbean should be among these non-synonymous SNPs. Based on the de novo assembly ( Supplementary Table 3 ), the genome-wide alignment of these scaffolds revealed considerable consistency in the overall genome organization between domesticated mungbean and its wild relative ( Supplementary Fig. 5 ). However, there was some degree (80–95%) of alignment block differentiation between wild and domesticated mungbean ( Supplementary Fig. 5 ). With 18,981 genes having a collinear relationship between the wild and domesticated mungbean, there was a recent peak of Ks frequency of the synteny blocks having a modal value at 0.01 (modal age of 1 million years ago (MYA)) ( Supplementary Table 10 ). The Ks values between VC1973A and V2984 were calculated using SNPs in coding sequences of V2984 , and consequently, its modal age was 1 MYA ( Supplementary Table 10 ). This is similar to the modal age between VC1973A and TC1966 , suggesting that allelic differences between cultivated and wild mungbean are similar to differences between cultivated mungbeans. Repetitive elements are known to be a major driving force behind plant evolution [26] . A higher proportion of repetitive elements is found in domesticated (50.1%) than in wild (46.9%) accession. While the other TEs were distributed equally in both species, Gypsy elements were more widely dispersed in domesticated mungbean accession ( Supplementary Table 4 ). Duplication history of legume genomes The subfamily Papilionoideae contains the majority of legume crops and the major model legume species, M. truncatula and L. japonicus . Members of this family shared an ancient whole-genome duplication (WGD) event ~58 MYA [7] , [8] , [9] , [10] , [11] before the family split into several major groups, the two largest being the warm-season millettioid and the cool-season Hologalegina clades, ~54 MYA [27] . Most of the legume crops within the millettioid clade, such as C. cajan and Phaseolus vulgaris , underwent no additional WGD events. However, the soybean genome underwent another round of WGD ~5–13 MYA, which resulted in its high chromosome number (2 n =4 x =40) and an increase of its genome size [10] , [28] . Comparison of 2,917 pairs of paralogous genes residing in duplicated collinear blocks within the mungbean genome revealed that the mungbean has experienced only one ancient WGD. There was a single major peak of Ks frequency of the synteny blocks with a modal value at 0.61 (modal age of 59 MYA), which is near the origin of the Papilionoideae ( Fig. 1c and Supplementary Table 10 ) [27] . In contrast, a recent peak at the Ks value of 0.07 (6.8 MYA) was detected from a pairwise comparison of homologues with no supporting collinearity of the genes, possibly because of recent small-scale duplications including tandem and ectopic duplication [29] ( Supplementary Fig. 6 ). Especially, tandem duplicates, which were searched by the homologous gene pairs located within 10 consecutive genes on the same chromosome, increased ~7–13 MYA, generating 252 tandem gene clusters with Ks peaks of ~0.06–0.12 ( Supplementary Fig. 7 ). The tandem duplicates were enriched for the following gene ontology category terms: ‘defence response’, ‘cell wall modification’, ‘secondary metabolic process’, ‘sulphate transport’, ‘recognition of pollen’, ‘transmembrane transport’ and ‘protein amino acid phosphorylation’ ( Supplementary Fig. 8 ). To understand more recent allopolyploidy in Vigna , we sequenced the genome of V. reflexo-pilosa var. glabra , which is known to be an allotetraploid (2 n =4 x =44; ref. 30 ). In total, 41,844 genes, almost twice the number of mungbean genes, were predicted based on A. thaliana and G. max proteins, in addition to the leaf transcriptome sequence of V. reflexo-pilosa var. glabra . The synteny blocks of V . reflexo - pilosa exhibited a recent peak with Ks values having a modal value at 0.07 (modal age of 6.8 MYA) and weak ancient traces consistent with the shared papilionoid WGD seen more clearly in V. radiata var. radiata and G. max ( Supplementary Table 10 and Fig. 1c ). Assuming that V . reflexo - pilosa var. glabra is allopolyploid, the divergence time of the donor species of the allopolyploid genome was estimated at 6.8 MYA. The genome comparison of V. radiata var. radiata with A. thaliana , C. arietinum , C. cajan , G. max , L. japonicus and M. truncatula revealed the presence of well-conserved macrosynteny blocks, although these blocks were highly dispersed among plant species with different numbers of chromosomes ( Supplementary Fig. 9 ). Given the closer relationship of Vigna to Glycine , most of the V. radiata var. radiata genes were found in genomic regions with synteny to G. max . Of the 18,378 genes on pseudochromosomes, 14,569 were located in 1,059 synteny blocks of orthologues or paralogues, which were used to determine the time of divergence between V. radiata and G. max . The frequency of median Ks of synteny blocks showed a peak with a modal value at 0.29 (modal age of 28 MYA; Fig. 2a–c and Supplementary Table 10 ). The non-collinear 3,807 genes on pseudomolecules, which may have been fractionated after the ancient WGD or duplicated at a small scale, were mostly enriched in the gene ontology categories of ‘defence response’ and ‘translation’ ( Supplementary Fig. 10 ). Comparisons of the estimated divergence times based on the peak Ks values showed that there was greater divergence between Vigna and Cajanus than between Vigna and Glycine , as expected. There were 11,853 mungbean genes in synteny with the C. cajan genome. The frequency of median Ks of synteny blocks showed the main peak having a modal value at 0.32 (modal age of 31 MYA) ( Fig. 2a,b,d and Supplementary Table 10 ). Divergence times estimated here were consistently larger than comparable estimates from chloroplast genes or non-genic regions [27] , [31] . Figure 2: Analysis of syntenic relationships in legumes within the millettioid clade. ( a ) Estimation of divergence times between V. radiata and C. cajan , and between V. radiata and G. max . ( b ) Visualization of chromosomal rearrangements among V. radiata var. radiata , G. max and C. cajan . Chromosomes among V. radiata var. radiata , C. cajan and G. max (A genome) are connected by red lines, and chromosomes between V. radiata var. radiata and G. max (B genome) are linked by blue lines. ( c ) Syntenic relationship between V. radiata and G. max ; the x -axis indicates chromosomal locations and the y -axis indicates Ks value. Each dot represents the location of a synteny block with its Ks median value, showing both conservation and chromosomal rearrangements of syntenic blocks. ( d ) Depiction of the syntenic relationship between V. radiata and C. cajan . Full size image Vigna speciation based on transcriptome analysis Speciation and domestication have involved substantial adaptations to various climates and cultural environments. Asian Vigna species (subgenus Ceratotropis) are morphologically and physiologically diverse, consistent with their distribution across South, Southeast and East Asia, extending from tropical regions to the Himalayan highlands [32] . Subgenus Ceratotropis has been divided into three taxonomic groups (Angulares, Ceratotropis and Aconitifoliae) based on its morphological characters such as seedling germination, floral size and growth habit [30] . From the de novo assembly of RNA-seq from leaf tissues of 22 accessions of 16 Asian Vigna species, representing each of these groups, as well as 1 African Vigna species ( V. subterranea ) and 1 Eurasian Vigna species ( V. vexillata ), we identified 1,121 shared orthologous loci using OrthoMCL [24] ( Supplementary Tables 11 and 12 ). Two phylogenetic analyses were conducted. (1) A Bayesian multispecies coalescent analysis (*BEAST [33] ) used 9 orthologous loci from 20 diploid Vigna species and the two homoeologous genomes of the polyploid, V. reflexo-pilosa as separate operational taxonomic units (OTU) based on the within-genome synteny relationship and the inter-genome synteny relationships with V. radiata var. radiata . This time-calibrated analysis also used the two reconstructed homoeologous genomes of G. max as outgroups and for calibration based on the ca. 19 MYA divergence of Vigna and Glycine estimated from chloroplast gene phylogenies [27] . (2) A maximum likelihood (ML) [34] analysis used 375 concatenated orthologous loci from 20 diploid Vigna accessions. The *BEAST and ML analyses both identified two clades with good support ( Fig. 3 , Supplementary Fig. 11 ), in agreement with a previously published chloroplast phylogeny [32] . The *BEAST and ML trees both placed V. subramaniana (which was not in the chloroplast analysis) as sister to V. radiata. Although there were several differences in some other clades appeared in all three phylogenies, which may be due to different sampling, the *BEAST analysis allowed relationships of the two homoeologous genomes of V. reflexo-pilosa to be traced. One was found to be closely related to diploid V. trinervia ( Fig. 3 ), in agreement with previous chloroplast results [32] and suggesting that V. trinervia or a close ally was the maternal progenitor of the allopolyploid. A maximum date for the polyploidy event of 0.09 MYA is given by the divergence between these two OTUs. The second homoeologous genome was found to be sister to the entire second diploid clade comprising the Angulares group; this topology and the much older divergence date (2.7 MYA) suggests that the diploid progenitor lineage has not been sampled, and may be extinct. Figure 3: Species tree for 22 Vigna accessions and close legume relative, G. max . Average divergence dates were depicted for the nodes estimated by a Bayesian MCMC method. The horizontal bars represent the 95% highest posterior density (HPD) interval at each node estimated by tested genes. The colour of the square on each node represents the posterior probability according to colour gradation from black (0) through blue (0.5) to red (1). The root divergence time was set to a 19 MYA between V. radiata var. radiata and G. max following the estimation of Lavin et al. [27] Full size image Genomic resources for mungbean breeding The development of molecular markers is critical for crop improvement programmes. Although molecular marker resources are limited for mungbean, there have been several efforts to identify the genomic regions related to domestication-related traits, including seed size and seed germination [35] . Moreover, molecular markers are important for integrating useful alleles of wild mungbean, such as bruchid resistance, into domesticated mungbean [36] ( Fig. 1a ). With our whole-genome sequencing and gene content data, a syntenic relationship was revealed by a comparative analysis with well-characterized G. max quantitative trait locus (QTLs) to provide important clues for the identification of mungbean QTLs. The synteny blocks of seed size/germination and bruchid resistance QTL regions matched the soybean synteny blocks containing simple sequence repeat (SSR) markers linked to seed weight and nematode resistance ( Fig. 1a ). Hence, our resequencing-derived wild-genotype-specific mungbean SNPs and the comparative genomic information may further facilitate a variety of molecular breeding activities and will ultimately assist the identification of the responsible genes for the corresponding traits. We also developed SSR markers using MISA software [37] , resulting in the identification of 200,808 SSRs from 1,544 scaffolds ( Supplementary Table 13 ). The number of tri-repeat unit SSRs, which were efficiently used for genotyping, was 17,898. The identification of molecular markers for the resistance against biotic and abiotic stresses is crucial. As previously reported, most resistance genes encode proteins with two core domains: nucleotide-binding sites (NBSs) and leucine-rich repeats (LRRs) [38] . A hidden Markov model (HMM) was established for each domain after a Pfam domain search. In mungbean, we found 73 LRR genes with NB-ARC domains, in which all of the NBS-LRR genes exhibited homology with known disease resistance genes in the UniProt database [39] . In addition, 19 of 464 LRR genes without NB-ARC domains were identified as genes for disease resistance and damage repair ( Supplementary Table 14 ). Our data revealed 30 SNP markers flanking resistance genes ( Supplementary Table 15 ). We constructed 421 Mb (80%) of the total estimated V. radiata var. radiata genome and identified 22,427 high-confidence protein-coding genes and 160 Vigna gene clusters. This is the first draft genome sequence within the genus Vigna . Together with the genome and transcriptome sequences of other Vigna species produced by this study, it will facilitate further genome research into the subgenus Ceratotropis. Genomic sequencing provided insights into the history of polyploidy in papilionoid legumes and within the genus Vigna . The signature of the ancient whole-genome duplication shared among papilionoid legumes such as Medicago , Lotus , Glycine and Cajanus — a peak in the age distribution of pairs of duplicated genes—was observed in Vigna species. The date of 59 MYA estimated from this distribution was consistent with previous estimates [40] , [41] . Bioinformatic separation of the allotetraploid (2 n =44) genome of V. reflexo-pilosa var. glabra into its constituent homoeologous subgenomes and their inclusion as separate taxa (A and B genomes) in a Bayesian species tree phylogeny allowed us to identify and date its origins. The allopolyploidy event occurred at maximum date of 0.09 MYA, with one diploid genome and the chloroplast genome donated by a close relative of V. trinervia and the second diploid genome from an unsampled member of a clade that included several species, among them V. minima , to which it has been considered to be related ( Fig. 4 ) [30] . Figure 4: Schematic illustration of allopolyploidization history of the V. reflexo - pilosa var. glabra . Red arrow indicates the putative date (maximum 0.09 MYA) of polyploidization event of V. reflexo-pilosa var. glabra . The number at each node represents the divergence time estimated by a Bayesian MCMC method. Full size image It has been suggested that the domestication and cultivation of mungbean was initiated in the northwest and far south of India 4,000–6,000 years ago, based on the geographical distribution of wild mungbean and archaeological records from India [5] . The domesticated mungbean is considered to have spread mainly throughout Southeast Asia and East Asia from India via different routes [42] . It is possible that the domesticated mungbean was imported from India to China via the Silk Road and subsequently spread to Southeast Asia. As we sampled only one accession of V. radiata var. sublobata in our study, we could not observe any population substructure in V. radiata var. sublobata , and we thus cannot determine whether there are V. radiata var. sublobata lineages more closely related to cultivated mungbean than the one we sampled, nor could we obtain evidence for multiple origins of the crop variety. Based on the Ks distribution, the divergence between the V. radiata var. radiata and V. radiata var. sublobata lineages sampled here and also between the V. radiata var. radiata ( VC1973A ) and V. radiata var. radiata ( V2984 ) occurred ~1 MYA, substantially predating domestication of mungbean (4,000–6,000 years ago) ( Supplementary Table 10 ). Similar findings about the divergence of wild lineages and their cultivated derivatives have been reported in other cultivated species, such as rice and soybean [43] , [44] . Mungbean is grown mostly in developing countries, which has delayed fundamental genome research. To date, because of the lack of genome sequence data for Vigna species, molecular breeding has not yet been fully implemented. The whole-genome sequence and the high-density genetic map give access to efficient SNP discovery and thus will boost genomics-assisted selection for mungbean improvement. Plant materials Twenty-two accessions of 18 Vigna species were used in this study, including the Asian domesticated species of black gram, mungbean, adzuki bean, rice bean, créole bean and moth bean, as well as the African domesticated species. In addition to those domesticated species, we combined the wild progenitors of black gram, mungbean, rice bean and créole bean. Instead of the wild progenitor of adzuki bean ( V. angularis var. nipponensis), V. nepalensis was included in this study as a variant of V. angularis var. nipponensis [45] , [46] . All of the species belong to the subgenus Ceratotropis (Asian Vigna ), with the exception of V. subterranea and V. vexillata which belongs to the subgenus Vigna (African Vigna ) and Plectotropis (Eurasian Vigna ), respectively. These accessions were collected from several national and international genebanks including Chai Nat Field Crops Research Center in Thailand, the National Agrobiodiversity Center in Korea, the National Institute of Agrobiological Sciences in Japan, the National Botanic Garden of Belgium in Belgium, the Australian Collections of Plant Genetic Resources in Australia, the International Center for Tropical Agriculture in Columbia, the International Livestock Research Institute in Kenya and the International Institute of Tropical Agriculture in Nigeria. These collected Vigna accessions have a diploid chromosome composition of 2 n =2 x =22, whereas V. reflexo-pilosa is an only allotetraploid Vigna species (2 n =4 x =44). Genome assembly We sequenced the mungbean genome by two NGS platforms, Illumina Hiseq2000 and GS FLX+, with five libraries of a 180-bp fragment, 5, 10, 40-kb mate-pairs and one single linear library. For genome assembly of V. radiata var. sublobata and V. reflexo-pilosa var. glabra , 180-bp fragment and 5-kb mate-pair libraries were sequenced by Illumina Hiseq2000. The reads produced by Illumina and GS FLX+ were assembled by using the software packages of ALLPATHS-LG [18] and newbler, respectively. The Newbler contigs were used to validate the assemblies of ALLPATHS-LG using megablast with an E -value cut-off of 1e−100. The not-matched and overlapped contigs were chopped into pseudo 5-kb mate-pair reads and then assembled again using ALLPATHS-LG. SSR were predicted based on ALLPATHS-LG assembled scaffolds through the software MISA ( http://pgrc.ipk-gatersleben.de/misa/misa.html ) with default parameters [37] . SNP/INDEL analysis and whole-genome alignment The short reads obtained from the V. radiata var. radiata ( V2984 ), Kyung-Ki Jaerae #5, and a V. radiata var. sublobata ( TC1966 ),wild mungbean, were used for SNP/INDEL analysis ( Supplementary Table 1 ). The mapping of total reads mapping was performed with NextGenMap [47] , followed by software Samtools version 0.1.19 for SNP/INDEL detection with following criteria: (1) minimum depth=5; (2) maximum depth=100; (3) all mapped reads support a homozygous genotype; (4) minimum mapping quality over 10 (ref. 48 ). SNP/INDELs were classified into genic and inter-genic regions. For those SNPs located in the CDS regions, we determined synonymous and non-synonymous changes after constructing the consensus sequences reflecting the position of SNPs. Furthermore, de novo assembled wild mungbean sequences were aligned against 11 pseudochromosomes of the cultivated mungbean by nucmer in the Mummer 3 software package [49] . The similarity between two genomes was calculated and visualized by mummerplot. Genetic map construction To construct a genetic map of mungbean, we sequenced an F 6 population of 190 RIL by Illumina Hiseq2000 through GBS [50] . Each individual genomic DNA was extracted and then fragmented by the ApeKI restriction enzyme. After a GBS adapter ligation and PCR, the fragments were validated by the Agilent Technologies Bio-analyzer 2100. The resulting sequence library was implemented in the Hiseq2000 sequencer. The output sequenced reads were aligned to the scaffolds by software Bowtie2 (ref. 51 ). The genotypes of 190 RILs in the population were retrieved using the samtools software package [48] . We collected polymorphic sites among 190 populations based on the set of the read depth thresholds of 5, and the quality score of 30 with allowance of 10 missing genotypes. They were grouped into 10-kb windows, and those windows showing an abnormal recombination were discarded. A polymorphic site with the lowest number of missing genotypes among populations was selected as a representative of each window. The 190 genotypes of the representative polymorphic sites were parsed and then carried onto Joinmap 4. Consequently, a total of 239 scaffolds were anchored to 11 pseudomolecules after constructing the genetic map of mungbean. Detection of transposable element and repeat masking Transposable elements were detected using the software packages LTR-harverst [21] and TransposonPSI ( http://transposonpsi.sourceforge.net/ ) with default parameters. Putative LTR-retrotransposons were annotated by LTR-digest [20] using a set of hmm signatures: PF03078.8, PF00385.17, PF01393.12, PF04094.7, PF07253.4, PF00552.14, PF05380.6, PF00077.13, PF08284.4, PF00078.20, PF07727.7, PF06815.6, PF06817.7, PF03732.10, PF00075.17, PF01021.12, PF04195.5, PF00692.12, PF00692.12 and PF00098. In addition, the hmm of AP_ty1copia and AP_ty3gypsy elements was built using their alignment information from GyDB [52] . Gene prediction and annotation The mungbean genome gene prediction was implemented using the MAKER pipeline [22] . Transcriptomes of mungbean from four different tissues of leaf, flower, root and pod were sequenced by Illumina Hiseq2000 and assembled by software Trinity [53] . We pooled de novo transcriptome assemblies and removed the redundant sequences by software CD-HIT [54] . For the gene prediction pipeline, we used the transcriptome assembly of mungbean, the protein sequences of G. max , and the complete protein sequences of Arabidopsis from Uniprot [39] . Once an initial prediction was made by the MAKER pipeline, its output results were used for training the software AUGUSTUS [55] model parameters for the accuracy of gene predictions. Using the trained model parameters of mungbean, we re-ran the prediction pipeline again against the repeat-masked mungbean scaffolds. A set of the resulting high-confident genes was annotated by software Interproscan5 (ref. 56 ). Furthermore, we used the leaf transcriptome of each species and the protein sequences of Arabidopsis and G. max for the successful prediction of genes in V. radiata var. sublobata and V. reflexo-pilosa var. glabra . TF classification We classified the TF families of the mungbean genome based on the TF classification rules as described in Lang et al. [57] Along with the V. radiata var. radiata protein sequences, the protein sequences of 8 plant genomes including 5 dicot plants ( A. thaliana, G. max, M. truncatula, C. cajan and C. arietinum ) and 3 monocots ( B. distachyon, Z. mays and O. sativa ) were classified into 101 TF families for further comparative analysis. If the Pfam annotation for plant genome was unavailable in the databases, we annotated the Pfam IDs using Interproscan5. Identification of non-coding RNA contents in mungbean genome Non-coding RNAs from transcriptome and genomic data were retrieved from database Rfam using software Infernal [58] , [59] . We made a subset of Rfam members among reference plants, A. thaliana , O. sativa , G. max and Vigna species. The sequences of Rfam sub-members were blasted against the transcriptome and genome sequences with the following threshold settings: number of alignments=5, E -value=1 and sequence similarity= 90%. Infernal were implemented on the matched regions including a flanking 50 bp and transcriptome assemblies to find significance of RNA secondary structure with an E -value cut-off of 0.001. Transcriptome assembly and Vigna speciation analysis The first leaf trifoliates of 22 Vign a accessions were harvested. Each of messenger RNA was extracted using TRIzol (Invitrogen, Life Technologies, Carlsbad, CA, USA) following the manufacturer’s instructions. All of the messenger RNA samples were converted into a 500 bp paired-end sequencing library to be suitable for a subsequent cluster generation using the TruSeq RNA Sample Preparation Kit (Illumina, San Diego, CA, USA). For RNA sequencing, the Illumina HiSeq2000 platform was used. The short reads were assembled by software Trinity [53] with default parameters. CDS from the assembly were retrieved by perl script and transcripts_to_best_scoring_ORFs.pl, which was included in Trinity. The redundancy of assembled coding sequences of 22 Vigna accessions was removed from software CD-HIT (ref. 54 ). The non-redundant assemblies of 22 Vigna species were clustered using Orthomcl software and found 1,121 shared orthologue loci. For the three Vigna species, V. radiata var. radiata , V. radiata var. sublobata and V. reflexo-pilosa var. glabra that was constructed into large scaffold by de novo genome assembly, we tried to determine the confident orthologues by synteny relationship with G. max and C. cajan . For the allopolyploid genomes, G. max and V. reflexo-pilosa var. glabra , we split the paralogous gene pairs as A and B genome using the recent Ks peak of within-genome synteny comparison and the synteny relationship against V. radiata ; using median Ks value of each synteny block, closer synteny block to V. radiata was set as A genome and the other was as B genome. Hence, two OTUs for each allopolyploid species were used to retrieve orthologues. The orthologues of A genome of G. max and V. reflexo-pilosa to V. radiata var. radiata , C. cajan and V. radiata var. sublobata were collected based on synteny relationship finding 173 loci. Finally, common 9 loci was retrieved between the transcriptome-based Orthomcl orthologues (1121 loci) and the synteny-based orthologues (173 loci). For estimation of the species tree, we implemented the Bayesian Markov Chain Monte Carlo (MCMC) analysis using the nine loci by the *BEAST option of the software package BEAST version 1.8 (ref. 33 ). We aligned the orthologues of nine loci using software Prank [60] . The analysis was initiated with random starting tree. Analysis consisted with two runs of MCMC with the length of chain being 50 million and the parameters logged at every 1,000 steps. For the substitution model, we run software Prottest [61] to select the model and we found JTT+G as the best model. For the clock model, we used relaxed clock model with log normally distributed uncorrelated rates. For root time calibration, we used ca. 19 MYA divergence of Vigna and Glycine estimated from chloroplast gene phylogenies of previous study. For ML tree, we used the 20 diploid Vigna transcriptome assemblies. Among the orthologous relationship from the Orthomcl result, we retrieved 375 orthologous loci that have one protein for each accession for the concatenation of the confident orthologous loci. The each locus was independently aligned using Prank software [60] . The concatenation of alignments was supplied to Phyml software for ML tree construction with 500 bootstraps [34] . Identification of disease resistance genes Using the Pfam annotations of the mungbean gene model, we retrieved the two core domains in which they are referred to as NBS and LRR. We used the Pfam IDs PF00931 for NBS domain and PF00560, PF07723, PF07725, PF12799, PF13306, PF13516, PF13504 and PF13855 for LRR domain. For each Pfam ID, the matched protein regions were retrieved and aligned again. The alignment results were converted into HMM of each domain by hmmbuild of software HMMER 3.0 ( http://hmmer.org ). Using our newly built HMM, NBS-LRR genes were searched using peptide sequences of mungbean by hmmsearch of software HMMER 3.0. The functions of the matched peptide within NBS and LRR domains were predicted by BLASTP analysis against Uniprot database [39] . Analysis of whole-genome duplication The whole-genome duplication and allopolyploidization of V. radiata , V. reflexo-pilosa and G. max were estimated using the collinearity within each genome. The protein sequences of each genome were initially self-blasted to determine a homologous relationship with an E -value threshold of 1e −10 . The collinearity based on the peptide locations in the genome was calculated by software MCScanX with default parameters [62] . Using the perl script, add_ka_and_ks_to_collinearity.pl included in MCScanX package, we calculated Ks values of the homologues within collinearity blocks. The median of Ks values was considered to be a representative of the collinearity blocks. The divergence times were estimated using the two different rates of 5.17 and 6.1 synonymous substitutions per synonymous site every 1 billion years [10] , [63] . Accession codes. The mungbean genome assembly, gene models, genetic marker information, annotations, and other related files have been deposited in GenBank/EMBL/DDBJ under the accession code JJMO00000000 . How to cite this article: Kang, Y. J. et al. Genome sequence of mungbean and insights into evolution within Vigna species. Nat. Commun. 5:5443 doi: 10.1038/ncomms6443 (2014).